Active control of electromagnetically induced transparency analogue in terahertz metamaterials Recently reported metamaterial analogues of electromagnetically induced transparency enable a unique route to endow classical optical structures with aspects of quantum optical systems. This method opens up many fascinating prospects on novel optical components, such as slow light units, highly sensitive sensors and nonlinear devices. In particular, optical control of electromagnetically induced transparency in metamaterials promises essential application opportunities in optical networks and terahertz communications. Here we present active optical control of metamaterial-induced transparency through active tuning of the dark mode. By integrating photoconductive silicon into the metamaterial unit cell, a giant switching of the transparency window occurs under excitation of ultrafast optical pulses, allowing for an optically tunable group delay of the terahertz light. This work opens up the possibility for designing novel chip-scale ultrafast devices that would find utility in optical buffering and terahertz active filtering. Electromagnetically induced transparency (EIT) is a quantum interference effect that occurs in three-level atomic systems and gives rise to a sharp transparency window within a broad absorption spectrum [1] . This effect markedly modifies the dispersive properties of an otherwise opaque medium that can lead to slow light phenomena and enhanced nonlinear effects. However, the demands of stable gas lasers and low temperature environment severely hamper the implementation of EIT in chip-scale applications. Recently, analogues of EIT-like behaviour in classical systems, such as coupled resonators [2] , [3] , electric circuits [4] and plasmonic structures [5] , [6] , [7] , [8] , [9] , [10] , [11] , [12] , [13] , [14] , [15] , [16] , have attracted enormous interest. These artificial structures possess EIT-like resonances due to Fano-type linear destructive interference [17] , [19] , but avert the scathing experimental requirements of quantum optical implementations. In particular, plasmonic analogues of EIT based on metamaterial structures, including cut wires (CWs), fishnets and split-ring resonators (SRRs), highlight the realization of bulk EIT analogues because of their effective medium characteristics. Their giant group refractive index and enhanced nonlinear properties have shown great promise in developing novel devices, such as slow light photonic components, integrated chip scale buffers, highly sensitive sensors or rulers and electromagnetically induced absorbers [20] , [21] , [22] , [23] . For practical applications, it is highly desirable that the group velocity of electromagnetic waves be actively controlled. This would resemble the true atomic EIT system where a pump beam is used to control the populations in the dipole-allowed state and the meta-stable state, and consequently the dispersion and group velocity of light. For this purpose, an active metamaterial is a promising candidate. Previous studies in the area of active metamaterials have shown various modulation schemes to control the properties of metamaterial-based devices [24] , [25] , [26] , [27] , [28] , [29] , [30] , [31] . In particular, optical tuning of metamaterials has attracted growing interest in the terahertz regime due to its ultrafast modulation speed and on-to-off switching capability [26] , [27] , [28] , [29] , [30] . However, so far the EIT effect in most metamaterials can only be tuned passively by varying the geometrical parameters of the resonator structures [32] , [33] , [34] , [35] , [36] , [37] , [38] . Only cryogenic-temperature-dependent EIT metamaterials have been reported recently [39] . In this article, we demonstrate, for the first time to our knowledge, active control of terahertz waves in classical EIT metamaterials at room temperature by integrating photoactive silicon (Si) islands into functional unit cells. An on-to-off active control of the EIT resonance is demonstrated by optical pump-terahertz probe (OPTP) measurements. Theoretical calculations and numerical simulations attribute this modulation to a change in the damping rate of the dark mode caused by the increased conductivity of the Si islands under photoexcitation. This work is a clear demonstration of an optically active classical analogue of the quantum EIT phenomena in metamaterials. The active tuning of group delay and group refractive index in particular may have promising applications in terahertz wireless communications. It may also inspire interest in developing electrical and mechanically tunable EIT metamaterials, resulting in a wide range of novel compact slow light devices. Design and characterization of the EIT metamaterial The unit cell of the EIT metamaterial consists of a CW and two SRRs, with Si islands positioned in their gaps, as shown in Fig. 1a . As the resonances of CW and SRR are both determined primarily by their geometrical dimensions and the size of the subwavelength unit cell ensures that the terahertz waves do not diffract at normal incidence, thus the EIT metamaterial array behaves as an effective medium. The metamaterial structure was fabricated on a Si-on-sapphire wafer comprised of 500-nm-thick undoped Si film and 495-μm-thick sapphire substrate with an image shown in Fig. 1b . The fabrication of the metamaterial sample began with patterning of Si islands by reactive ion etching, followed by deposition of 200-nm-thick aluminium that forms the CW and the SRR-pair patterns. The fabricated sample array occupies an area of 10×10 mm. 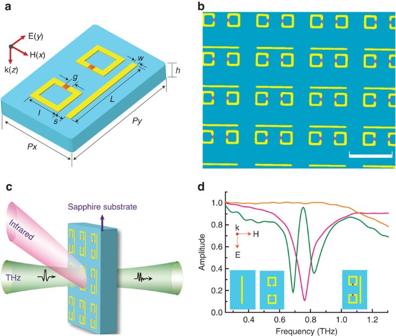Figure 1: Experimental design and measured transmission spectra. (a) Schematic of the unit cell. The geometrical parameters are:L= 85,l=29,s=7,w=5,h=495,g=5,Px=80 andPy=120 μm, respectively. (b) Microscopic image of the fabricated metamaterial. Scale bar, 100 μm. (c) Experimental schematic of the optical pump-terahertz probe measurements of the EIT metamaterial. (d) Measured amplitude transmission spectra of the sole-CW (pink), SRR-pair (orange) and the EIT metamaterial sample (olive). The insets in (d) are the structural geometries of the sole-CW, SRR-pair and the EIT metamaterial samples from left to right, respectively, with the polarization illustration. Figure 1: Experimental design and measured transmission spectra. ( a ) Schematic of the unit cell. The geometrical parameters are: L = 85, l =29, s =7, w =5, h =495, g =5, Px =80 and Py =120 μm, respectively. ( b ) Microscopic image of the fabricated metamaterial. Scale bar, 100 μm. ( c ) Experimental schematic of the optical pump-terahertz probe measurements of the EIT metamaterial. ( d ) Measured amplitude transmission spectra of the sole-CW (pink), SRR-pair (orange) and the EIT metamaterial sample (olive). The insets in ( d ) are the structural geometries of the sole-CW, SRR-pair and the EIT metamaterial samples from left to right, respectively, with the polarization illustration. Full size image An electro-optic time-resolved OPTP system, as illustrated in Fig. 1c , was used to carry out the measurements [30] (see Methods). The 2.5-mm diameter terahertz beam was collimated on the metamaterial array with electric field parallel to the CW. An optical pump beam (50 fs, 1.35 mJ per pulse at 800 nm with a 1-kHz repetition rate) with a spot diameter of 10 mm enables a uniform excitation aperture for the terahertz transmission. A bare sapphire wafer identical to the sample substrate serves as a reference. The measured transmission through the EIT metamaterial sample and the blank reference has a time extent of the terahertz pulse scans of 12 ps to remove the Fabry–Perot reflections from the rear facet without causing distortion in the main terahertz pulse. The normalized transmission spectrum is defined as (ref. 40 ), where and are Fourier transforms of the measured time-domain terahertz pulses of the sample and reference, respectively. To clarify the underlying mechanism of the EIT effect, we fabricated and measured three sets of samples. The first sample consists of a CW array, the second consists of an SRR-pair array and the third (the EIT metamaterial sample) consists of both the CW and the SRR-pair. The measured amplitude transmissions of the first (CW only) and the second samples (SRR-pair only) are shown in Fig. 1d . The CW resonator array shows a typical localized surface plasmon (LSP) resonance at 0.74 THz whereas the SRR-pair that supports an inductive–capacitive (LC) resonance at the same frequency is inactive due to the perpendicular orientation of the incident electric field. Thus, the CW resonator and the SRR-pair serve as the bright and dark modes, respectively, for perpendicular electric field excitation. In the EIT sample the CW is directly excited by the incident electric field along the CW. The near field coupling between the CW and the SRR-pair excites the LC resonance in the SRRs. The destructive interference between the LSP and LC resonances leads to a sharp transparency peak in a broad absorption background at 0.74 THz, as illustrated in Fig. 1d . Next, the transmission property of the EIT sample under different optical excitations is investigated. The transmitted time-domain pulses and the corresponding normalized amplitude spectra in frequency domain are shown in Fig. 2a,b , respectively. When there is no photoexcitation, a pronounced subsidiary wave packet is observed following the main pulse in the time domain, which is a characteristic of a wave packet with slow group velocity. In the corresponding frequency domain spectrum, an EIT peak is observed between two resonance dips with a transmission amplitude of 85% at 0.74 THz. As the excitation power of the pump beam is gradually increased from 25 to 1,000 mW, the subsidiary wave packet decreases in magnitude, and the corresponding transmission undergoes a strong modulation, as illustrated in Fig. 2a,b , respectively. When the pump power is >1,000 mW, the transparency window gradually decreases to 50% and the EIT peak vanishes. With the maximum photoexcitation of 1,350 mW, the time-domain subsidiary packet completely disappears and only a single broad LSP resonance dip as low as 43% is observed in the transmission spectrum, thus completing an on-to-off EIT peak modulation. In this modulation process, the recovery time of the excited carriers in Si is ~1 ms, which is not ultrafast in this sample. However, the active EIT metamaterial may achieve the ultrafast dynamical tuning characteristic if the intrinsic Si is replaced with a semiconductor film of a short carrier life time [41] . 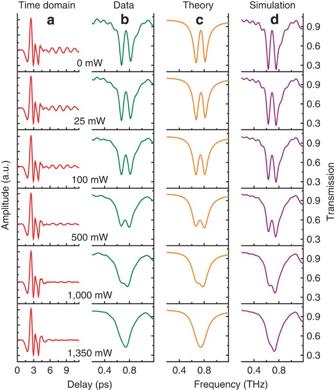Figure 2: Active control of the transparency window. (a) Measured transmitted time-domain signals and (b) corresponding normalized Fourier transformed amplitude spectra. (c) Theoretical fitting results for various damping rates. (d) Numerical simulation results of normalized spectra of the EIT metamaterial with different conductivities of the Si islands. Figure 2: Active control of the transparency window. ( a ) Measured transmitted time-domain signals and ( b ) corresponding normalized Fourier transformed amplitude spectra. ( c ) Theoretical fitting results for various damping rates. ( d ) Numerical simulation results of normalized spectra of the EIT metamaterial with different conductivities of the Si islands. Full size image Theoretical calculations To explore the physical origin of the active EIT behaviour, the widely used coupled Lorentz oscillator model is adapted to analyze the near field interaction between the two elements in the EIT metamaterial unit cell [5] . Similar to the three-level system in quantum EIT, this model involves a ground state |0 and two excited states |1 and |2 . The dipole-allowed transition |0 →|1 and the dipole-forbidden transition |0 →|2 correspond to the LSP bright mode resonance in the CW and the LC dark mode resonance in the SRR-pair, respectively. The transition between |1 and |2 corresponds to the coupling between the CW and the SRR-pair, which introduces destructive interference between pathways |0 →|1 and |0 →|1 →|2 →|1 , resulting in a strong suppression of loss and a very large dispersion within a narrow frequency band. In the EIT metamaterials, this interference can be analytically described by the coupled Lorentz oscillator model shown as where x 1 , x 2 , γ 1 and γ 2 are the amplitudes and the damping rates of the bright and dark modes, respectively. ω 0 =2π×0.74 THz and ( ω 0 + δ ) are resonance frequencies of the bright and dark modes, respectively. κ is the coupling coefficient between the two resonators and g is a geometric parameter indicating the coupling strength of the bright mode with the incident electromagnetic field E . According to equation (1), we express the susceptibility of one EIT metamaterial unit cell by δ , κ , γ 1 and γ 2 (ref. 5 ). Thus, the susceptibility of the EIT metamaterial layer with a thickness d is expressed as As the metamaterial layer is much thinner than the wavelength of the terahertz wave, the far-field transmission of the EIT sample can be approximately related to the near field susceptibility as (see Methods). where c is the light velocity in vacuum and n Sap =3.42 is the refractive index of the sapphire substrate [42] . Figure 2c shows the analytical fit using equation (2) to the measured amplitude transmission spectra under different photoexcitation fluences, exhibiting very good agreement with the measurements and simulations ( Fig. 2d ). The fitting parameters with increasing pump power are plotted in Fig. 3 . It is observed that δ , γ 1 and κ do not change significantly with increased photoexcitation fluence, whereas the damping rate of the dark mode γ 2 increases markedly from 0.025 THz (half of γ 1 ) without pump to 0.271 THz (four times γ 1 ) at 1,350 mW of pump power. Thus, it can be concluded from Fig. 3 that the active modulation of the EIT resonance arises from the change in the damping rate of the dark mode. Photoexcitation enhances the loss in the SRR-pair and hampers the destructive interference between the bright and dark modes. At the highest pump power of 1,350 mW, γ 2 becomes large enough to completely suppress the dark mode excitation, which eventually leads to the disappearance of the EIT resonance peak. 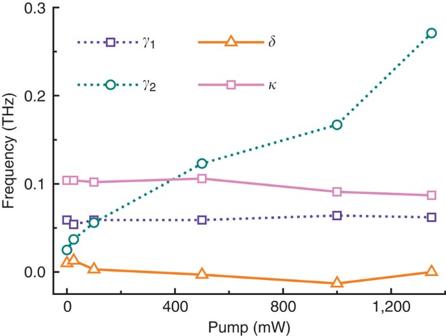Figure 3: Excitation-dependent behaviour of fitting parameters. δ,γ1,γ2andκare the parameters used in the far-field transmission fitting of the EIT metamaterial under different optical pump powers. The unit ofKis THz2. Figure 3: Excitation-dependent behaviour of fitting parameters. δ , γ 1 , γ 2 and κ are the parameters used in the far-field transmission fitting of the EIT metamaterial under different optical pump powers. The unit of K is THz 2 . Full size image Numerical simulations The correlation between the carrier excitations and the deterioration of the dark mode is numerically investigated using the commercial finite-integration package CST Microwave Studio TM . In the simulation, the sapphire substrate was treated as a lossless dielectric with ε Sap =11.7 and Al was modelled as a lossy metal with a conductivity of 3.72×10 7 S m −1 . The conductivity of the Si islands at the SRR gaps was varied to simulate the effect of optical excitation, that is, the carrier excitation in the Si islands [27] . As the optical power increased from 0 to 1,350 mW, the Si conductivity ( σ Si ) increased from 160 to 4,050 S m −1 . The simulation results shown in Fig. 2d are in good agreement with the measurements. The dark mode degradation can be understood by analyzing the distribution of the simulated normally polarized electric field at the EIT resonance frequency. 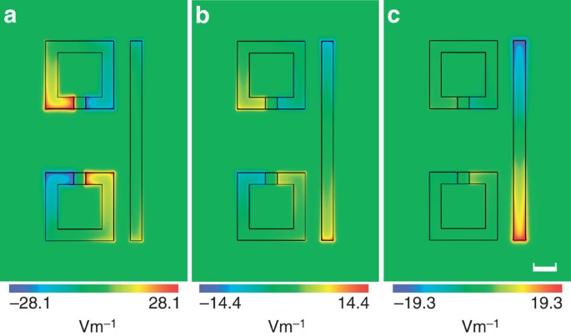Figure 4: Electric field distribution normal to the EIT layer. The corresponding optical excitations are (a) 0 mW (σSi=160 S m−1), (b) 1,000 mW (σSi=3,000 S m−1) and (c) 1,350 mW (σSi=4,050 S m−1), respectively. Scale bar, 10 μm. Figure 4 shows these distributions at σ Si =160, 3,000 and 4,050 S m −1 , corresponding to different photoexcitation power leading to pronounced EIT peak, EIT disappearance and only LSP resonance, respectively. Without optical pump, the Si islands are mainly dielectric and the SRR resonators exhibit very small damping. The figure shows that the electric field is primarily focused around the SRR gap, whereas the electric field in the CW is completely suppressed, which is the characteristic of a typical EIT effect [5] . On photoexcitation, the conductivity of the Si islands gradually increases, resulting in a redistribution of the electrical field in the EIT structures. This is verified in Fig. 4b where the SRR and the CW are both excited when the pump power is up to 1,000 mW. Furthermore, at 1,350 mW excitation ( σ Si =4,050 S m −1 ), the electric field in the SRR gaps is completely suppressed and the field distribution is localized at the plasmon resonance of the CW array. Clearly, the origin of the EIT resonance modulation essentially comes from the optically tunable conductivity of the Si islands due to the photodoping effect. Figure 4: Electric field distribution normal to the EIT layer. The corresponding optical excitations are ( a ) 0 mW ( σ Si =160 S m −1 ), ( b ) 1,000 mW ( σ Si =3,000 S m −1 ) and ( c ) 1,350 mW ( σ Si =4,050 S m −1 ), respectively. Scale bar, 10 μm. Full size image The slow light capability of the EIT phenomena has been widely discussed in previous works [1] , [5] , [8] . The ability to actively control the slow light capability will enable both scientific research frontiers and upcoming optical techniques. The measurement of the slow light effect is represented by the group delay (Δ t g ) of the terahertz wave packet through the sample, instead of normally used group refractive index ( n g ) [3] , [39] . The use of Δ t g is more relevant to represent the slow light capability of a device and more importantly, Δ t g retrieval does not require the effective thickness of the sample, which is difficult to define owing to the influence of the substrate on the EIT resonance. The difference in Δ t g through the EIT metamaterial and vacuum with the same thickness is retrieved from their complex transmissions (by Fourier transform) at various photoexcitations, as shown in Fig. 5 . Notably, the group delays retrieved from the measurements ( Fig. 5a ) and the calculation ( Fig. 5b ) match very well. The wave packet shown in Fig. 5a with central frequency 0.74 THz is delayed by 5.74 ps (including the propagation in the substrate), which is equivalent to the time delay of a 1.72-mm distance of free space propagation. However, as the photoexcitation increases to 1,350 mW, the EIT metamaterial array gradually loses its slow light characteristic, finally turning into a typical LSP group delay feature. To verify the practicality of the tunable EIT metamaterial, an estimated value of n g could be actively tuned from 91 without optical pump to 10.5 at 500 mW photoexcitation at 0.74 THz with an assumption of 6 μm effective sample thickness. This thickness was assumed as the normally polarized electric field amplitude falls below 1/ e value of that at the metamaterial surface. The highest n g representing the slow light tunability is comparable to the previously reported group index values in EIT metamaterials [2] , [3] , [5] , [7] , [8] , [10] , [12] , [39] . Most significantly, the active tuning of n g demonstrated in this work may directly lead to compact, optically controllable slow light devices. 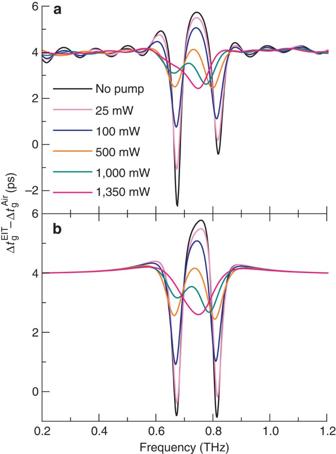Figure 5: Optically tunable active group delay. Group delays retrieved from (a) measured transmission spectra and (b) theoretical calculations according to equation (2) under different photoexcitations.andare the group delays through the active EIT metamaterial and vacuum with the same thickness, respectively. Figure 5: Optically tunable active group delay. Group delays retrieved from ( a ) measured transmission spectra and ( b ) theoretical calculations according to equation (2) under different photoexcitations. and are the group delays through the active EIT metamaterial and vacuum with the same thickness, respectively. Full size image In summary, by incorporating Si islands into the metamaterial unit cell, we have demonstrated an optically reconfigurable EIT effect in planar metamaterials functioning at terahertz frequencies. Theoretical analysis based on the coupled Lorentz oscillator model and far field OPTP measurements verifies that this novel active EIT switching is attributed to the suppression of the dark mode LC resonance. The distribution of electrical field normal to the EIT layer reveals that the dark mode could be controlled by optically tuning the conductivity of the integrated Si islands. In addition, the optical control of the group delay in the EIT metamaterial is also demonstrated both from experimental measurements and theoretical calculations. The optically active tuning of EIT metamaterials may open up avenues for designing active slow light devices, ultrasensitive sensors and nonlinear devices. OPTP measurements Under normal incidence, the metamaterials were characterized using an OPTP spectrometer. The output near-infrared laser beam (50 fs, 3.2 mJ pulse at 800 nm with a 1-kHz repetition rate) was split into two parts with one being used for terahertz generation detection and the other for optical excitation of the metamaterial samples through a variable neutral density attenuator. The pump beam has a beam diameter of 10 mm, much larger than that of the focused terahertz spot (~3 mm) at the sample, providing uniform excitation of the metamaterial array. The variation in the pump-probe time delay was implemented using a motion stage through changing the pump beam optical path. Under various pump powers, the transmitted terahertz pulses through the EIT metamaterials and the blank sapphire reference were measured in the time-domain, thus recording the time-varying electric field of the impulsive terahertz radiation. The transmission amplitude and phase spectra were directly obtained by performing fast Fourier transformation of the time-domain signals and normalized to those of the reference. Theoretical derivation of the far-field transmission In the OPTP measurements, the far-field transmissions through the EIT sample and reference were obtained. The schematic of the transmission measurements are shown in Fig. 6 . 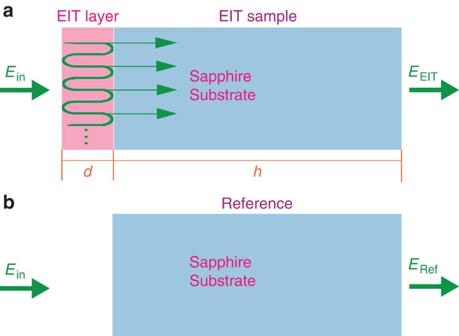Figure 6: Schematic of transmission measurements. Transmission through (a) EIT metamaterial sample and (b) reference blank substrate.Einis the incident terahertz electric field whileEEITandERefare the transmitted terahertz electric fields through the metamaterial and reference, respectively. The thicknesses of the metafilm,d, and substrate,h, are 700 nm and 495 μm respectively. The olive lines in the metafilm illustrate the Fabry–Perot interference. The measured amplitude transmission | t ( ω )| can be expressed as Figure 6: Schematic of transmission measurements. Transmission through ( a ) EIT metamaterial sample and ( b ) reference blank substrate. E in is the incident terahertz electric field while E EIT and E Ref are the transmitted terahertz electric fields through the metamaterial and reference, respectively. The thicknesses of the metafilm, d , and substrate, h , are 700 nm and 495 μm respectively. The olive lines in the metafilm illustrate the Fabry–Perot interference. Full size image where is the transmission at the first air–sapphire interface of the reference sample, which can be directly obtained from the Fresnel coefficients. is the Fabry–Perot interference transmission of the EIT layer, which could be expressed as where is the refractive index of the EIT metafilm and n Sap =3.42 is that of the lossless sapphire substrate. c is the light velocity in vacuum. As d ~700 nm is very thin compared with the wavelengths of the terahertz wave, the d →0 limit of equation (3) presented below was adapted to evaluate the measured far-field transmission How to cite this article: Gu, J. et al . Active control of electromagnetically induced transparency analogue in terahertz metamaterials. Nat. Commun. 3:1151 doi: 10.1038/ncomms2153 (2012).